PHF20 regulates NF-κB signalling by disrupting recruitment of PP2A to p65 Constitutive NF-κB activation in cancer cells is caused by defects in the signalling network responsible for terminating the NF-κB response. Here we report that plant homeodomain finger protein 20 (PHF20) maintains NF-κB in an active state in the nucleus by inhibiting the interaction between PP2A and p65. We show that PHF20 induces canonical NF-κB signalling by increasing the DNA-binding activity of NF-κB subunit p65. In PHF20 overexpressing cells, the termination of tumour necrosis factor-induced p65 phosphorylation is impaired whereas upstream signalling events triggered by tumour necrosis factor are unaffected. This effect strictly depends on the interaction between PHF20 and methylated lysine residues of p65, which hinders recruitment of PP2A to p65, thereby maintaining p65 in a phosphorylated state. We further show that PHF20 levels correlate with p65 phosphorylation levels in human glioma specimens. Our work identifies PHF20 as a novel regulator of NF-κB activation and suggests that elevated expression of PHF20 may drive constitutive NF-κB activation in some cancers. NF-κB is a member of a family of transcription factors that control the expression of a multitude of critical genes that regulate cell survival, proliferation, apoptosis and immune responses [1] , [2] , [3] . Given the pivotal role of NF-κB signalling downstream of a multitude of receptors for a variety of ligands, such as tumour necrosis factor (TNF), interleukin 1 (IL-1) and toll-like receptor (TLR) ligands, NF-κB signalling must be engaged temporally and spatially in check by well orchestrated negative feedback loops to prevent excessive activation [4] , [5] . On the other hand, defects in the regulation of NF-κB pathways contribute to a variety of pathological diseases, including autoimmune disease and cancer [6] , [7] , [8] , [9] , [10] , [11] , implicating the existence of a strong association between loss of normal regulation of NF-κB and cancer. Discovered over a series of monumental steps, well-established negative regulators include the ubiquitin-editing proteins A20 and CYLD as well as the quintessential NF-κB inhibitor IκBs [12] , [13] , [14] , [15] , [16] . Despite the progress, the negative regulation and/or aberrant dysregulation of active NF-κB in the nucleus is largely unexplored. Plant homeodomain finger protein 20 (PHF20, also termed glioma-expressed antigen 2) was initially discovered as an autoantibody in patients suffering from glioblastoma [17] . Subsequently, it was found that PHF20 was abundantly expressed in various cancers [18] , [19] , [20] , suggesting that PHF20 could have a role in cancer development. Although little is known about its cellular function, recent studies have revealed that PHF20 is a component of H4K16 histone acetyltransferase ‘male absent on the first’ (MOF) complex, which can bind to methylated Lys residue on the histone tail [21] , [22] . Moreover, PHF20-deficient mice demonstrated defective transcriptional activation of H4K16 target genes [23] , suggesting that PHF20 is a potent transcriptional activator by a epigenetic-based mechanism. Interestingly, a recent report has shown that a Tudor domain in PHF20 can also associate with p53 through dimethylated Lys residues, leading to stabilization of p53 (ref. 24 ). Therefore, it is assumed that, in addition to histone methylation, PHF20 may also target methylated non-histone proteins such as transcription factor p53 or NF-κB for transcriptional activation. Herein, we describe a novel role of PHF20 in NF-κB signalling: PHF20 promotes NF-κB transcriptional activity by interacting with p65 in a methylation-dependent manner. We found that the interaction of PHF20 with methylated p65 contributes to persistent p65 phosphorylation by disrupting the recruitment of phosphatase PP2A. Moreover, we observe significant correlations between PHF20 and p65 phosphorylation in sets of clinical glioma tissues. These results establish a novel function of PHF20 as a key protein in the positive feedback mechanism to constitutively maintain NF-κB in a default active state in cancer development. PHF20 acts as a positive regulator of NF-κB signalling Based on its domain structure, PHF20 is predicted to function as a regulator of transcription factor. In an initial screening using an activation profiling array, we found that NF-κB was one of the positive transcription factors identified in cells with ectopic expression of PHF20 (data not shown). To systematically assess the involvement of PHF20 in NF-κB signalling, we first examined the transcriptional activity of NF-κB in 293/IL-1R/TLR4 cells stably overexpressing IL-1R and TLR4. Overexpression of PHF20 resulted in a remarkable increase of NF-κB luciferase activity in response to various stimuli, including TNF, IL-1β, lipopolysaccharide (LPS) and a DNA-damaging agent (etoposide) ( Fig. 1a ). Consistently, PHF20 knockdown led to a significantly reduction of NF-κB reporter activity induced by each of these stimuli ( Fig. 1b ). Such observations thus indicate that PHF20 is able to upregulate NF-κB activation in a canonical pathway. Confirming this suspicion, NF-κB activation mediated by the IKKs and adaptor proteins RIP1, TRAF2, TRAF6 and MyD88 also was significantly enhanced by PHF20 ( Fig. 1c ). 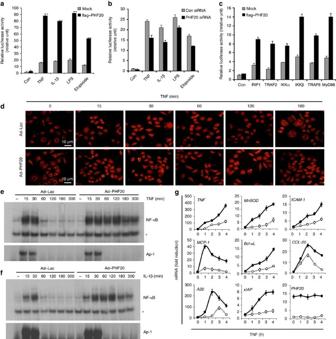Figure 1: PHF20 is a positive regulator of NF-κB signalling. (a,b) 293/IL-1R/TLR4 cells were transiently transfected with p2xNF-κB-Luc and pRSV-β-gal with expression plasmids of the flag–PHF20 or PHF20 short interfering RNA (150 pmol). After 24 h of transfection, cells were treated for 6 h with TNF (15 ng ml−1), IL-1β (10 ng ml−1), LPS (1 μg ml−1) and etoposide (20 μM). (c) 293/IL-1R/TLR4 cells were transiently transfected with indicated expression plasmids along with p2xNF-κB-Luc and pRSV-β-gal. Luciferase assays were performed as described in Methods, and the activity of each sample was normalized according to β-galactosidase activity. Each columns shows mean±s.e. of at least three independent experiments.*P<0.05, compared with mock-transfected cells (Student’st-test) (d–g) HeLa cells were infected with either rAd–Lac or rAd–PHF20 for 24 h, and then treated with TNF or IL-1β for indicated times. (d) Subcellular localization of p65 was analysed by immunofluorescence confocal microscopy with a rabbit anti-p65 antibody (red). Scale bar, 10 μM. (e,f) Electrophoretic mobility shift assay was performed as described in Methods. AP-1-binding activity serves as a positive control. * indicates nonspecific binding to NF-κB probe. (g) mRNA expression levels of NF-κB target genes (TNF,MnSOD,ICAM-1,MCP-1,Bcl-xL,CCL-20,A20 and xIAP) were measured by real-time RT–PCR (, rAd–Lac;, rAd–PHF20). The data represent results from three independent experiments (mean±s.e. of triplicate). Figure 1: PHF20 is a positive regulator of NF-κB signalling. ( a,b ) 293/IL-1R/TLR4 cells were transiently transfected with p2xNF-κB-Luc and pRSV-β-gal with expression plasmids of the flag–PHF20 or PHF20 short interfering RNA (150 pmol). After 24 h of transfection, cells were treated for 6 h with TNF (15 ng ml −1 ), IL-1β (10 ng ml −1 ), LPS (1 μg ml −1 ) and etoposide (20 μM). ( c ) 293/IL-1R/TLR4 cells were transiently transfected with indicated expression plasmids along with p2xNF-κB-Luc and pRSV-β-gal. Luciferase assays were performed as described in Methods, and the activity of each sample was normalized according to β-galactosidase activity. Each columns shows mean±s.e. of at least three independent experiments. *P <0.05, compared with mock-transfected cells (Student’s t -test) ( d – g ) HeLa cells were infected with either rAd–Lac or rAd–PHF20 for 24 h, and then treated with TNF or IL-1β for indicated times. ( d ) Subcellular localization of p65 was analysed by immunofluorescence confocal microscopy with a rabbit anti-p65 antibody (red). Scale bar, 10 μM. ( e , f ) Electrophoretic mobility shift assay was performed as described in Methods. AP-1-binding activity serves as a positive control. * indicates nonspecific binding to NF-κB probe. ( g ) mRNA expression levels of NF-κB target genes ( TNF,MnSOD,ICAM-1,MCP-1,Bcl-xL,CCL-20,A20 and xIAP ) were measured by real-time RT–PCR ( , rAd–Lac; , rAd–PHF20). The data represent results from three independent experiments (mean±s.e. of triplicate). Full size image Furthermore, in HeLa cells with overexpression of PHF20, prolonged nuclear retention of p65 and p50 occurred after treatment with TNF in comparison with the untreated control cells ( Fig. 1d and Supplementary Fig. S1 ). Notably, in cells with expression of PHF20, we observed prolonged NF-κB-DNA binding induced by both TNF ( Fig. 1e ) and IL-1β ( Fig. 1f ). Importantly, AP-1-binding activities in response to TNF or IL-1β were not affected by PHF20. Consistently, expression of the NF-κB target genes induced by TNF was substantially enhanced in cells overexpressed with PHF20 ( Fig. 1g ). Furthermore, such enhanced expression of the NF-κB target genes by PHF upon TNF treatment was drastically abolished in p65 null (p65−/−) mouse embryonic fibroblasts (MEFs), in contrast to that in wild-type MEFs ( Supplementary Fig. S2 ), confirming that the effect of PHF20 on NF-κB activation is p65-dependent. Together, data from this part demonstrate that PHF20 is able to upregulate NF-κB activity by promoting its nuclear retention and NF-κB–DNA binding. PHF20 does not affect upstream events of NF-κB signalling To gain further insight into the molecular mechanisms underlying PHF20-mediated NF-κB activation, we next examined the phosphorylation and degradation of IκBα. Upon TNF treatment, IκBα was phosphorylated and degraded with the similar degree and kinetics in rAd–PHF20-infected cells, as compared with rAd–Lac-infected cells ( Fig. 2a ). Consistently, TNF-induced IKK activity was not affected by PHF20 overexpression ( Fig. 2c ), indicating that upregulation of TNF-induced NF-κB signalling by PHF20 is independent of IKK. This conjecture also seems to be consistent with the above observation that PHF20 does not interfere with p65 nuclear translocation ( Fig. 1d ). Moreover, treatment of cells with TNF led to immediate interaction of IKK-γ with hyper-ubiquitinated RIP1, and consistently the extent and duration of TNF-induced ubiquitinated RIP1–IKK interaction was not affected by PHF20 overexpression ( Fig. 2d ), confirming that PHF20 likely functions downstream of IKK activation and IκBα degradation in simulating NF-κB activation. 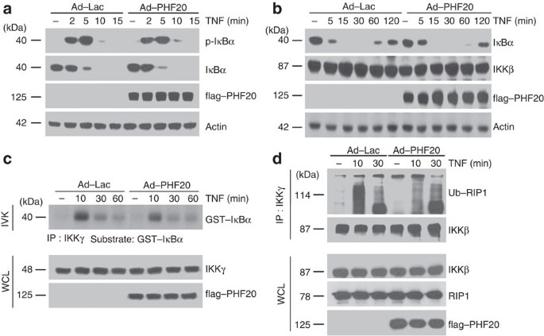Figure 2: PHF20 does not affect the upstream signalling events of NF-κB activation. HeLa cells were infected with either rAd–Lac or rAd–flag–PHF20 for 24 h, and then cells were treated with TNF for indicated times. (a,b) Whole-cell lysates were immunoblotted with indicated antibodies. (c) Cell extracts were subjected to immunoprecipitation with anti-IKK-γ antibody, and its activity was assessed by immune complex kinase assay as described in Methods (upper panel). The efficiency of immunoprecipitant of IKK complex was confirmed by immunoblotting with anti-IKKγ antibody (lower panel). Relative densities of phosphorylated GST–IκBα were obtained by densitometry for corresponding IKK-γ at each lane. (d) Cell extracts from each sample were subjected to immunoprecipitation with anti-IKKγ antibody. Immunoprecipitates were analysed by immunoblotting with indicated antibodies. A total of 1% of the cell extract volume (WCL) from each sample was used as input control. Figure 2: PHF20 does not affect the upstream signalling events of NF-κB activation. HeLa cells were infected with either rAd–Lac or rAd–flag–PHF20 for 24 h, and then cells were treated with TNF for indicated times. ( a,b ) Whole-cell lysates were immunoblotted with indicated antibodies. ( c ) Cell extracts were subjected to immunoprecipitation with anti-IKK-γ antibody, and its activity was assessed by immune complex kinase assay as described in Methods (upper panel). The efficiency of immunoprecipitant of IKK complex was confirmed by immunoblotting with anti-IKKγ antibody (lower panel). Relative densities of phosphorylated GST–IκBα were obtained by densitometry for corresponding IKK-γ at each lane. ( d ) Cell extracts from each sample were subjected to immunoprecipitation with anti-IKKγ antibody. Immunoprecipitates were analysed by immunoblotting with indicated antibodies. A total of 1% of the cell extract volume (WCL) from each sample was used as input control. Full size image PHF20 induces sustained phosphorylation of p65 To further probe the role of PHF20 in the nuclear step of NF-κB signalling, we next examined whether PHF20 affects the phosphorylation status of the p65 subunit of NF-κB, an essential event in nuclear NF-κB signalling. Notably, phosphorylation of p65 was markedly prolonged in rAd–PHF20-infected cells in response to TNF, whereas only transient p65 phosphorylation was found in control cells ( Fig. 3a , top). Moreover, we found that such effect by PHF20 was specific to p65, based on the results that TNF-induced phosphorylation of ERK and JNK was not affected by PHF20 ( Fig. 3a , third and fifth rows). To further confirm the generality of our observation, we generated a single vector-inducible system by tebufenozide ( teb ). This system displayed tight regulation of teb -dependent PHF20 expression in a dose- and time-dependent manner without any detectable basal level ( Supplementary Fig. S3a , b ). Important to note, the overexpression of PHF20 using this inducible system also caused persistent phosphorylation of p65, but not of ERK and JNK ( Fig. 3c ). Furthermore, we also observed that different expression levels of PHF20 with different dosage of teb well correlated with the extent of the TNF-induced persistent p65 phosphorylation ( Supplementary Fig. S3b ) as well as NF-κB reporter activity ( Supplementary Fig. S3c ). Consistently, knocking down PHF20 led to a more evident reduction of TNF-induced NF-κB reporter activity in teb -treated cells harbouring high levels of PHF20 expression, compared with the control cells ( Supplementary Fig. S4 ). 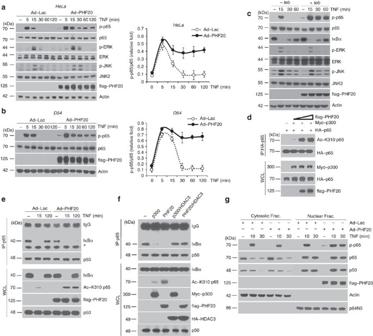Figure 3: Failure to terminate TNF-induced phosphorylation of p65 by PHF20. (a,b) HeLa and D54 cells were infected with either rAd–Lac or rAd–flag–PHF20 for 24 h, and then cells were treated with TNF for indicated times. Whole-cell lysates were immunoblotted with indicated antibodies (left). Relative density was obtained by densitometry of the corresponding immunoblot data. Data are from one representative of three independent experiments (mean±s.e. of triplicate, (right). (c)Teb-on PHF20 HEK293 cells were incubated with or withoutteb(25 μM) for 12 h, and then further treated with TNF for indicated times. Whole-cell lysates were immunoblotted as ina. (d) HEK293 cells were co-transfected with the expression plasmids of HA-p65, Myc-p300 and different amounts of flag–PHF20. Immunoprecipitates were prepared with anti-HA antibody and immunoblotted with anti-Acetyl-p65-Lys310 antibodies. Whole-cell lysates were immunoblotted as ina. (e) HeLa cells were infected with either rAd–Lac or rAd–flag–PHF20, which was followed by TNF treatment for indicated times. After the immunoprecipitation with anti-p65 antibody, immunoprecipitated IκBα was detected by immunoblotting with anti-IκBα antibody (top first row). Co-immunoprecipitated p50 serves as a positive control (top second row). Whole-cell lysates were immunoblotted as ina. The asterisk indicates nonspecific bands for anti-IκBα antibody. (f) HEK293 cells were co-transfected with the indicated expression plasmids, and followed by TNF treatment for 2 h. Immunoprecipitates were prepared with anti-p65 antibody and immunoblotted as ine. (g) HeLa cells were infected with either rAd–Lac or rAd–flag–PHF20, and followed by TNF treatment for indicated times. Cytosolic and nuclear fractions were obtained, and immunoblot was performed as ina. Figure 3: Failure to terminate TNF-induced phosphorylation of p65 by PHF20. ( a,b ) HeLa and D54 cells were infected with either rAd–Lac or rAd–flag–PHF20 for 24 h, and then cells were treated with TNF for indicated times. Whole-cell lysates were immunoblotted with indicated antibodies (left). Relative density was obtained by densitometry of the corresponding immunoblot data. Data are from one representative of three independent experiments (mean±s.e. of triplicate, (right). ( c ) Teb -on PHF20 HEK293 cells were incubated with or without teb (25 μM) for 12 h, and then further treated with TNF for indicated times. Whole-cell lysates were immunoblotted as in a . ( d ) HEK293 cells were co-transfected with the expression plasmids of HA-p65, Myc-p300 and different amounts of flag–PHF20. Immunoprecipitates were prepared with anti-HA antibody and immunoblotted with anti-Acetyl-p65-Lys310 antibodies. Whole-cell lysates were immunoblotted as in a . ( e ) HeLa cells were infected with either rAd–Lac or rAd–flag–PHF20, which was followed by TNF treatment for indicated times. After the immunoprecipitation with anti-p65 antibody, immunoprecipitated IκBα was detected by immunoblotting with anti-IκBα antibody (top first row). Co-immunoprecipitated p50 serves as a positive control (top second row). Whole-cell lysates were immunoblotted as in a . The asterisk indicates nonspecific bands for anti-IκBα antibody. ( f ) HEK293 cells were co-transfected with the indicated expression plasmids, and followed by TNF treatment for 2 h. Immunoprecipitates were prepared with anti-p65 antibody and immunoblotted as in e . ( g ) HeLa cells were infected with either rAd–Lac or rAd–flag–PHF20, and followed by TNF treatment for indicated times. Cytosolic and nuclear fractions were obtained, and immunoblot was performed as in a . Full size image Next, we examined the effect of PHF20 on p65 acetylation based on the sequential link between phosphorylation and acetylation in the regulation of NF-κB function [25] , [26] . As expected, overexpression of PHF20 drastically enhanced p65 acetylation in cells with co-transfection of p300 acetylatransferase ( Fig. 3d ), as well as TNF-induced interaction between endogenous p65 and p300 ( Supplementary Fig. S5 ). As a reversible acetylation of p65 governs IκBα binding to display nucleocytoplasmic shuttling properties of NF-κB complex [27] , we thus examined whether such an enhanced acetylation status of p65 by PHF20 might affect its interaction with IκBα. Notably, overexpression of PHF20 resulted in persistent dissociation of p65 and IκBα for up to 2 h upon TNF treatment, despite the fact that comparable amount of total IκBα levels were expressed in the cell ( Fig. 3e ). In addition, such an interrupted interaction between p65 and IκBα in the presence PHF20 was restored by co-expression of HDAC3 ( Fig. 3f ), which has an essential role in p65 deacetylation through a physical interaction [27] , [28] . We further assessed whether the phosphorylation of p65 by PHF20 occurred in the nucleus. It is noteworthy that TNF-induced transient phosphorylations of p65 at 10 min in both of cytosolic and nuclear fractions were not affected by PHF20. In contrast, TNF-induced p65 phosphorylations at 30 min by PHF20 were only present in the nuclear fraction, despite the fact that comparable amounts of p65 and p50 were translocated in each sample ( Fig. 3g ). These observations clearly suggest that in the nucleus the potency of PHF20 to interrupt the assembly of p65 with IκBα through enhanced p65 phosphorylation and subsequently its acetylation contributes to prolong NF-κB response. Recent reports indicated that PHF20 was phosphorylated at Ser291 and Ser265 by Akt/PKB [29] , [30] . Here, we further assessed whether the phosphorylation status of PHF20 is functionally involved in its effect on p65 phosphorylation. In control cells, PHF20 was phosphorylated on Ser291 but not Ser265 ( Supplementary Fig. S6a ). Upon TNF treatment, overexpression of non-phosphorylatable mutant of PHF20 (PHF20/S291A) also enhanced persistent p65 phosphorylation as well as NF-κB reporter activity, but to a less extent than the wild-type PHF20 or PHF20/S265A ( Supplementary Fig. S6b , c ). Similar effects of wild-type PHF20 and PHF20/S291A on the p65 phosphorylation were also found in teb -inducible system ( Supplementary Fig. S6d ), suggesting that Akt/PKB-mediated phosphorylation of PHF20 partly contribute to its regulatory effect on p65 phosphorylation. PHF20 interacts with methylated lysine residues of p65 The ability of members of Tudor domain subfamily to bind methylated protein substrates or histone tails has been well documented [21] , [22] , [24] . Thus, we next attempted to investigate the role of p65 methylation in the PHF20-mediated NF-κB activation. Pretreatment with a broad methylation inhibitor, 5′-deoxy-5′-methylthioadenosine (MTA), markedly inhibited NF-κB luciferase activity ( Fig. 4a ) and NF-κB-DNA binding ( Fig. 4b ) in response to TNF, without affecting phosphorylation and degradation of IκBα ( Fig. 4c ). Remarkably, MTA pretreatment in cells overexpressing PHF20 almost completely inhibited TNF-induced luciferase activity and NF-κB-DNA binding. Consistently, MTA pretreatment abrogated the phosphorylation and acetylation of p65 in cells with PHF20 overexpression ( Fig. 4d ). However, transient p65 phosphorylations until 10 min were not affected by MTA pretreatment in control cells ( Fig. 4c , third row), suggesting that cellular context of methylation does not involve in early stage of TNF-induced p65 phosphorylation. 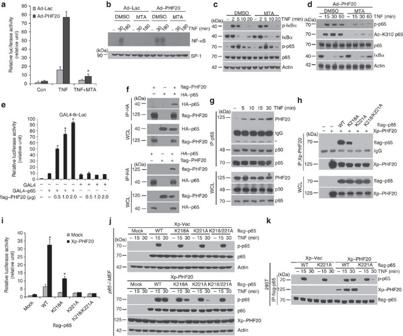Figure 4: PHF20 activates NF-κB by interacting with Lys-methylated p65 (a) HeLa cells were infected with either rAd–Lac or rAd–flag–PHF20 and transfected with an NF-κB-responsive reporter plasmid. After 24 h, cells were pretreated with MTA (1 mM) for 1 h, and treated with TNF for 6 h. Luciferase assays were performed as inFig. 1a. (b) HeLa cells were infected with either rAd–Lac or rAd–flag–PHF20. After 24 h, cells were pretreated with MTA, followed by TNF for indicated times. Electrophoretic mobility shift assay was performed as inFig. 1e. (c) HeLa cells were pretreated with MTA, followed by TNF treatment. Whole-cell lysates were analysed by immunoblot with indicated antibodies. (d) HeLa cells were infected with rAd–flag–PHF20. After 24 h, cells were pretreated with MTA, followed by TNF treatment. Whole-cell lysates were analysed by immunoblot with indicated antibodies. (e) HEK293 cells were co-transfected with indicated GAL4 constructs with or without PHF20 plasmids. After 24 h, GAL4-tk-Luc reporter activity was measured as described ina. (f) HEK293 cells were co-transfected with indicated tagged PHF20 and p65 plasmids for 24 h. Immunoprecipitates were prepared with anti-flag or anti-HA antibody, and immunoblotted with indicated antibodies. (g) HeLa cells were treated with TNF for indicated times. After immunoprecipitation with anti-p65 antibody, immunoprecipitated PHF20 was detected with anti-PHF20 antibody (top first row). Co-immunoprecipitated p50 serves as a positive control (top second row). The asterisk indicates nonspecific bands for anti-PHF20 antibody. (h,i) HEK293 cells were co-transfected with Xp-tagged PHF20 along with either mock or flag-tagged various forms of p65, followed by TNF for 10 min. (h) After immunoprecipitation with anti-Xp antibody, immunoprecipitated p65 was measured by immunoblotting with anti-flag antibody. (i) Luciferase assay was performed as described in a. (j) p65−/− MEFs were co-transfected as described inhand followed by TNF for indicated times. Whole-cell lysates were analysed by immunoblot with indicated antibodies. (k) HEK293 cells were co-transfected with Xp-tagged PHF20 along with flag-tagged p65 (WT or K221A) as described inhand, followed by TNF for indicated times. Immunoprecipitates were prepared with anti-flag antibody and immunoblotted with indicated antibodies. Each column shows mean±s.e. of at least three independent experiments (Student’st-test).*P<0.05, compared with TNF-treated group (a), GAL4–p65 only-transfected group (e) or wild-type p65-transfected group (i). Figure 4: PHF20 activates NF- κ B by interacting with Lys-methylated p65 ( a ) HeLa cells were infected with either rAd–Lac or rAd–flag–PHF20 and transfected with an NF-κB-responsive reporter plasmid. After 24 h, cells were pretreated with MTA (1 mM) for 1 h, and treated with TNF for 6 h. Luciferase assays were performed as in Fig. 1 a. ( b ) HeLa cells were infected with either rAd–Lac or rAd–flag–PHF20. After 24 h, cells were pretreated with MTA, followed by TNF for indicated times. Electrophoretic mobility shift assay was performed as in Fig. 1 e. ( c ) HeLa cells were pretreated with MTA, followed by TNF treatment. Whole-cell lysates were analysed by immunoblot with indicated antibodies. ( d ) HeLa cells were infected with rAd–flag–PHF20. After 24 h, cells were pretreated with MTA, followed by TNF treatment. Whole-cell lysates were analysed by immunoblot with indicated antibodies. ( e ) HEK293 cells were co-transfected with indicated GAL4 constructs with or without PHF20 plasmids. After 24 h, GAL4-tk-Luc reporter activity was measured as described in a . ( f ) HEK293 cells were co-transfected with indicated tagged PHF20 and p65 plasmids for 24 h. Immunoprecipitates were prepared with anti-flag or anti-HA antibody, and immunoblotted with indicated antibodies. ( g ) HeLa cells were treated with TNF for indicated times. After immunoprecipitation with anti-p65 antibody, immunoprecipitated PHF20 was detected with anti-PHF20 antibody (top first row). Co-immunoprecipitated p50 serves as a positive control (top second row). The asterisk indicates nonspecific bands for anti-PHF20 antibody. ( h , i ) HEK293 cells were co-transfected with Xp-tagged PHF20 along with either mock or flag-tagged various forms of p65, followed by TNF for 10 min. ( h ) After immunoprecipitation with anti-Xp antibody, immunoprecipitated p65 was measured by immunoblotting with anti-flag antibody. ( i ) Luciferase assay was performed as described in a. ( j ) p65−/− MEFs were co-transfected as described in h and followed by TNF for indicated times. Whole-cell lysates were analysed by immunoblot with indicated antibodies. ( k ) HEK293 cells were co-transfected with Xp-tagged PHF20 along with flag-tagged p65 (WT or K221A) as described in h and, followed by TNF for indicated times. Immunoprecipitates were prepared with anti-flag antibody and immunoblotted with indicated antibodies. Each column shows mean±s.e. of at least three independent experiments (Student’s t -test). *P <0.05, compared with TNF-treated group ( a ), GAL4–p65 only-transfected group ( e ) or wild-type p65-transfected group ( i ). Full size image To investigate the direct involvement of p65 in the transactivation of NF-κB by PHF20, we tested whether PHF20 stimulates GAL4–p65-dependent transcription on GAL4-driven reporter (GAL4-tk-Luc). Notably, co-expression of PHF20 specifically enhanced GAL4-tk transcriptional activity by p65 overexpression ( Fig. 4e and Supplementary Fig. S7 ), suggesting that such transactivation of NF-κB by PHF20 is achieved through its functional association with p65. The physical interaction between PHF20 and p65 was further verified in co-immunoprecipitation analysis ( Fig. 4f ). Furthermore, we also found the endogenous association of PHF20 with p65 in HeLa cells, and such interaction was gradually enhanced upon TNF treatment ( Fig. 4g ). To identify which domain of PHF20 was responsible for its interaction with p65, we generated several deletion mutants of PHF20 ( Supplementary Fig. S8a ). Similar co-immunoprecipitation experiments showed that only PHF20 containing a mutant Tudor2 domain (PHF20Δ69) was able to interact with p65, similar to the wild-type PHF20 protein. On the other hand, all other PHF20 mutants with deletion of the Tudor2 domain failed to precipitate together with p65, indicating that the Tudor2 domain of PHF20 is critical for the interaction with p65. As the p65/p50 heterodimer is the primary mediator of NF-κB transcriptional activity in the canonical pathway induced by TNF [31] , we next examined whether PHF20 also interacts with p50, another key NF-κB protein. As expected, co-immunoprecipitation experiments showed that PHF20 also interacted with p50 to a similar extent as did p65 ( Supplementary Fig. S9a ). However, TNF treatment of p65−/− MEFs resulted in no detectable binding of PHF20 with p50, as evident in wild-type MEFs ( Supplementary Fig. S9b ), which indicates that PHF20 interacts with the NF-κB complex (p65/p50) via p65. It has been demonstrated that p65 was monomethylated on lysine 218 (K218) and dimethylated on lysine221 (K221) [32] ; we next examined whether lysine methylation of p65 was required for the interaction with PHF20. To address this issue, constructs encoding wild-type p65 or three K-A mutants, in which lysine was substituted by alanine, were transiently transfected with PHF20 into HEK293 cells. In the co-immunoprecipitation assay, K221A or K218/221A mutant of p65 completely abolished the interaction with PHF20, whereas K218A mutant only partially affected the interaction in comparison with WT–p65 ( Fig. 4h ). Of note, the ability of PHF20 to NF-κB activation was drastically impaired in cells with the K221A or K218/221A mutant of p65, compared with that with wild-type p65 ( Fig. 4i ). These results suggest that K221 methylation of p65, which is required for its interaction with PHF20, has a critical role in PHF20-mediated NF-κB activation. To confirm the methylation-dependent interaction between PHF20 and p65, the full-length PHF20 with point mutations (W97A and/or Y103A) of the methyl-lysine-binding cage within the Tudor2 domain were generated, as reported earlier [24] . In the context of full-length proteins, the W97A– and/or Y103A–PHF20 markedly decreased the ability of the interaction with p65, compared with that of wild-type PHF20 ( Supplementary Fig. S10a ). Consistent with these results, the W97A– and/or Y103A–PHF20 failed to upregulate TNF-induced NF-κB activation, whereas PHF20 mutant containing a Tudor2 domain (PHF20Δ69) enhanced the activation of NF-κB by TNF, to a degree similar to that obtained with wild-type PHF20 ( Supplementary Fig. S10b ). To further scrutinize whether K221 methylation is directly involved in p65 phosphorylation mediated by PHF20, we re-expressed three mutants of p65 or wild-type p65 in p65−/− MEF. Interestingly, no difference was found for TNF-induced p65 phosphorylation among in p65−/− MEF reconstituted with either WT or three methylation-deficient p65, without the co-expression of PHF20 ( Fig. 4j , top). In contrast, a strikingly different result was obtained in cells with PHF20 overexpression: reconstitution with mutant p65 (K221A− or K218/221A) that was unable to bind PHF20 abolished the persistent p65 phosphorylation in response to TNF ( Fig. 4j , bottom). To further confirm the above observations, we compared the ability of PHF20 to regulate p65 phosphorylation in the immunoprecipitants of WT and K221A mutant of p65. Consistently, the phosphorylation of K221A–p65 at a later time point was only faintly detectable compared with that of WT–p65, whereas the transient phosphorylation at 15 min was unaffected by PHF20 overexpression ( Fig. 4k ). Taken together, these results clearly indicate that Lys221 site of p65 is indeed essential for the function of PHF20 in amplifying TNF-induced NF-κB activation via persistent phosphorylation of p65. PHF20 interrupts the recruitment of PP2A to p65 To understand how PHF20 prolongs TNF-induced p65 phosphorylation, we tested the possibility that PHF20 may disrupt the function of protein phosphatase(s). To do so, we examined the effects of four candidate phophatases, including PP1, PP2A, PP4 and WIP1, which were known to negatively regulate NF-κB signalling via dephosphorylation [33] , [34] , [35] , [36] . In this screen, particularly, PHF20-mediated upregulation of p65 phosphorylation was efficiently inhibited by PP2A, but not other three phosphatases tested ( Fig. 5a ). These results thus raised the possibility that PHF20 may specifically target PP2A, hence inducing persistent p65 phosphorylation in response to TNF. To validate this hypothesis, the possibly opposing effects of PHF20 on the TNF-driven NF-κB reporter activity when PP2A is silenced or overexpressed were investigated. Importantly, PP2A knockdown effectively prevented the enhancing effect of PHF20, which occurs upon stimulation by TNF ( Fig. 5b ). Consistently, overexpression of PP2A was able to abolish TNF-induced NF-κB activation, whereas its inhibitory effect was competitively antagonized by PHF20 overexpression depending on the expression level ( Fig. 5c ). We also observed that overexpression of PHF20 had a marginal effect on the upregulated p65 phosphorylation in cells with PP2A knockdown after TNF exposure ( Fig. 5d ). These results collectively indicate that PP2A is indeed a key phosphatase responsible for controlling p65 phosphorylation status through which PHF20 regulates NF-kB activation. 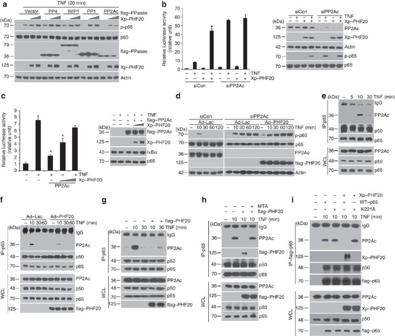Figure 5: PHF20 limits recruitment of PP2A to p65 in response to TNF. (a) HEK293 cells were co-transfected with flag-tagged phosphatases (PP1, PP2Ac, PP4 or WIP1) and Xp-tagged PHF20 plasmids, and followed by TNF for 20 min. Whole-cell lysates were analysed by immunoblot with indicated antibodies. (b) HEK293 cells were transfected with either 150 pmol of scramble (control) or PP2Ac short interfering RNA (siRNA) along with mock or Xp-tagged PHF20.*P<0.05, compared with TNF-treated group in scramble siRNA-transfected cells (mean±s.e. of triplicates). (c) HEK293 cells were co-transfected flag-tagged PP2Ac with different amounts of Xp-tagged PHF20. After 48 h, cells were treated with TNF for 6 h as indicated, and luciferase assays were performed as described inFig. 1a. Transfection efficiency of either overexpression or knock downed expression was confirmed by immunoblotting with indicated antibodies (right).*P<0.05, compared with TNF-treated group in mock-transfected cells (mean±s.e. of triplicates). (d) HeLa cells were transfected with either scramble (control) or PP2Ac siRNA along with rAd–Lac or rAd–flag–PHF20 and followed by TNF for the indicated times. Whole-cell lysates were analysed by immunoblot with indicated antibodies. (e) HeLa cells were treated with TNF for indicated times. After immunoprecipitation with anti-p65 antibody, co-immunoprecipitated PP2Ac was detected by immunoblotting with anti-PP2Ac antibody (top row). (f) HeLa cells were infected with either rAd–Lac or rAd–flag–PHF20 as described indand were treated with TNF for indicated times. Cells were lysed and immunoprecipitated with anti-p65 and immunoblotting was performed ine. (g) Similar experiments as described infusing flag-tagged PHF20 expression plasmid in HEK293 cells. HEK293 cells were transfected with either mock or flag-tagged PHF20, followed by TNF for 10 min in the absence or presence of MTA. (h) Similar experiments as described inf, with immunoprecipitation (IP) using anti-p65 antibody. (i) HEK293 cells were co-transfected with Xp-tagged PHF20 along with either flag-tagged WT or K221A mutant of p65 and followed by TNF for 10 min. Similar experiments as described inf, with IP using anti-flag antibody. Figure 5: PHF20 limits recruitment of PP2A to p65 in response to TNF. ( a ) HEK293 cells were co-transfected with flag-tagged phosphatases (PP1, PP2Ac, PP4 or WIP1) and Xp-tagged PHF20 plasmids, and followed by TNF for 20 min. Whole-cell lysates were analysed by immunoblot with indicated antibodies. ( b ) HEK293 cells were transfected with either 150 pmol of scramble (control) or PP2Ac short interfering RNA (siRNA) along with mock or Xp-tagged PHF20. *P <0.05, compared with TNF-treated group in scramble siRNA-transfected cells (mean±s.e. of triplicates). ( c ) HEK293 cells were co-transfected flag-tagged PP2Ac with different amounts of Xp-tagged PHF20. After 48 h, cells were treated with TNF for 6 h as indicated, and luciferase assays were performed as described in Fig. 1 a. Transfection efficiency of either overexpression or knock downed expression was confirmed by immunoblotting with indicated antibodies (right). *P <0.05, compared with TNF-treated group in mock-transfected cells (mean±s.e. of triplicates). ( d ) HeLa cells were transfected with either scramble (control) or PP2Ac siRNA along with rAd–Lac or rAd–flag–PHF20 and followed by TNF for the indicated times. Whole-cell lysates were analysed by immunoblot with indicated antibodies. ( e ) HeLa cells were treated with TNF for indicated times. After immunoprecipitation with anti-p65 antibody, co-immunoprecipitated PP2Ac was detected by immunoblotting with anti-PP2Ac antibody (top row). ( f ) HeLa cells were infected with either rAd–Lac or rAd–flag–PHF20 as described in d and were treated with TNF for indicated times. Cells were lysed and immunoprecipitated with anti-p65 and immunoblotting was performed in e . ( g ) Similar experiments as described in f using flag-tagged PHF20 expression plasmid in HEK293 cells. HEK293 cells were transfected with either mock or flag-tagged PHF20, followed by TNF for 10 min in the absence or presence of MTA. ( h ) Similar experiments as described in f , with immunoprecipitation (IP) using anti-p65 antibody. ( i ) HEK293 cells were co-transfected with Xp-tagged PHF20 along with either flag-tagged WT or K221A mutant of p65 and followed by TNF for 10 min. Similar experiments as described in f , with IP using anti-flag antibody. Full size image Earlier study reported that p65 could directly interact with PP2A in an in-vitro assay [36] . We found that, in response to TNF, endogenous interaction of p65 with PP2A was readily detectable in HeLa cells ( Fig. 5e ) or HEK293 cells ( Fig. 5g ), which peaked at 10 min post TNF treatment. Important to note, such a TNF-dependent p65/PP2A interaction was drastically abolished by either infection of rAd–PHF20 in HeLa cells ( Fig. 5f ) or transient transfection of flag–PHF20 in HEK293 cells ( Fig. 5g ). Surprisingly, treatment with MTA completely restored the impaired p65–PP2A interaction caused by PHF20 ( Fig. 5h , top). In the same blot, TNF-induced interaction between p65 and PHF20 was prevented by MTA treatment ( Fig. 5h , second panel), suggesting that the methylation-dependent interaction of PHF20 with p65 blocks the recruitment of PP2A into p65. To confirm the above notion, we repeated the experiments in cells with co-expression of wild-type or K221A mutant of p65 lacking the ability to interact with PHF20. Compared with wild-type p65, TNF-induced interaction between K221A–p65 and PP2A was not affected by PHF20 overexpression ( Fig. 5i ). These observations collectively suggest that PHF20 is able to effectively abolish the interaction of p65 with its phosphatase, PP2A, thus leading to persistent phosphorylation of p65 and promotion of NF-κB activation. Correlation of PHF20 and phospho-p65 levels in gliomas To understand the pathological importance of our findings, we examined whether the PHF20-p-p65 axis discovered in our cellular model is also applicable to clinical glioma tumours. By analysing 36 glioma tissue specimens with immunohistochemical analysis, we found that, in agreement with early findings [37] , [38] , expression of p-p65, an indicator of NF-κB activation, was largely detected in the nucleus and its levels were strongly correlated with WHO tumour grades ( Fig. 6a and Table 1 ). Similarly, the immunopositive PHF20 was found in 94.4% (34 out of 36) of glioma specimens detected exclusively in the nucleus along with p-p65 expression ( Fig. 6a and Table 2 ). To test the interaction of PHF20 and p-p65 in vivo , we performed immunohistochemical staining using serially sectioned tissues, and observed that both PHF20 and p-p65 were colocalized in the nucleus ( Fig. 6b ). These data were further confirmed by immunofluorescent co-staining for PHF20 and p-p65 expression, and identifying their colocalization in glioma tissues expressing both proteins ( Fig. 6c ). Univariate analysis revealed that expression levels of PHF20 were significantly associated with pathological tumour grade ( P =0.003; Table 2 ). Indeed, in grade IV tumours 81% (17 out of 21) of specimens was found to have higher immunopositivity to PHF20. Furthermore, correlation analysis showed that PHF20 expression levels were significantly correlated with the p-p65 levels ( P =0.0018; Fig. 6d ). These clinical observations provide a possible link between PHF20 overexpression and p65 phosphorylation in human malignant gliomas, resulting in constitutive activation of NF-κB and consequent promotion of tumorigenicity in glioma cells. 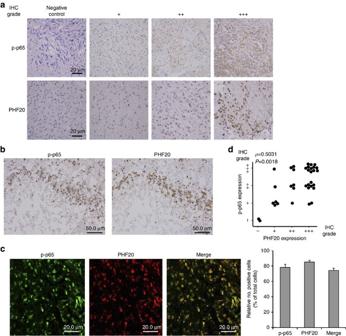Figure 6: p-p65 levels are associated with PHF20 expression in primary human glioma specimens. (a) Immunohistochemical staining of p-p65 and PHF20 in paraffin-embedded tissue specimens from 36 glioma patients. Negative control with exclusion of primary antibody. The intensity of histological staining grade was scored using a four-point scale: −, no staining, +, weak staining, ++ intermediate staining and +++ strong staining. Each representative case was shown (original magnification, × 400). Scale bar, 20 μm). (b,c) Representative image of colocalization between p-p65 and PHF20 expression in the nuclei of the glioma tumour cells. (b) Serial sections of tissues were prepared and stained simultaneously with anti-p-p65 and anti-PHF20 antibodies. Scale bars, 50 μm. (c) Immunofluorescence images of colocalization of p-p65 and PHF20 in glioma tissue specimen (grade IV, original magnification, × 600). Merge: the merge images represent the merging of p-p65 (green) and PHF20 (red) immunofluorescent staining (Scale bars: 20.0 μm). The percentage of cells with immunopositive staining was quantified by counting the number of positive cells by ImageJColocalization Plugin software at original magnification × 20 (mean±s.e. of triplicate, (right)). (d) Correlation between the expression levels of p-p65 and PHF20 were determined by theχ2test or linear-by-linear association in 36 collected human glioma samples (P=0.0018). Figure 6: p-p65 levels are associated with PHF20 expression in primary human glioma specimens. ( a ) Immunohistochemical staining of p-p65 and PHF20 in paraffin-embedded tissue specimens from 36 glioma patients. Negative control with exclusion of primary antibody. The intensity of histological staining grade was scored using a four-point scale: −, no staining, +, weak staining, ++ intermediate staining and +++ strong staining. Each representative case was shown (original magnification, × 400). Scale bar, 20 μm). ( b,c ) Representative image of colocalization between p-p65 and PHF20 expression in the nuclei of the glioma tumour cells. ( b ) Serial sections of tissues were prepared and stained simultaneously with anti-p-p65 and anti-PHF20 antibodies. Scale bars, 50 μm. ( c ) Immunofluorescence images of colocalization of p-p65 and PHF20 in glioma tissue specimen (grade IV, original magnification, × 600). Merge: the merge images represent the merging of p-p65 (green) and PHF20 (red) immunofluorescent staining (Scale bars: 20.0 μm). The percentage of cells with immunopositive staining was quantified by counting the number of positive cells by Image J Colocalization Plugin software at original magnification × 20 (mean±s.e. of triplicate, (right)). ( d ) Correlation between the expression levels of p-p65 and PHF20 were determined by the χ 2 test or linear-by-linear association in 36 collected human glioma samples ( P =0.0018). Full size image Table 1 Correlation between the histopathological tumour grading and expression of p-p65 in tissues of patients with glioma. Full size table Table 2 Correlation between the histopathological tumour grading and expression of PHF20 in tissues of patients with glioma. Full size table In this study, we report that PHF20, a protein with few known biological functions, is a novel positive regulator of NF-κB pathway that enhances and prolongs nuclear p65 phosphorylation in response to a variety of stimuli, including TNF or IL-1β. We have shown that PHF20 interacted with the methylated p65 (K218 and/or K221) and that the effect of PHF20 on NF-κB activation is dependent on p65 methylation. More importantly, such methylation-dependent interaction of PHF20 and p65 interrupts the recruitment of PP2A to p65 and thus maintains phosphorylated p65 in a default active state (as illustrated in Fig. 7 ). Therefore, these findings give rise to the possibility that PHF20 functions as a positive effector that causes constitutive NF-κB activation, as in the context of pathological conditions such as inflammation-linked cancer development. 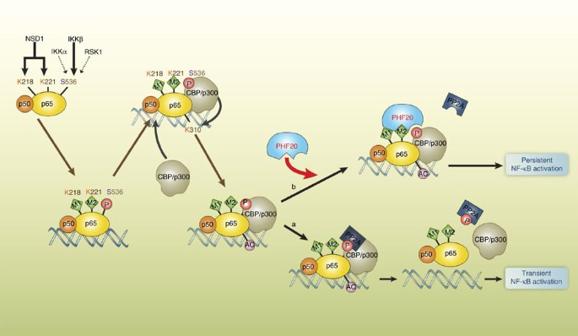Figure 7: Model for persistent activation of NF-κB by PHF20. It is known from the literature that NSD1 targets p65 for methylation on Lys218 and Lys221 residue functions to stabilize the formation of p65–DNA complex. p65 is also phosphorylated on Ser536 by various kinases, including IKKα, IKKβ or RSK1, which enhances its transactivation potential through recruiting histone acetyltransferase such as CBP and p300. (a) The recruitment of PP2A into phosphorylated p65 ensures that the NF-κB response maintains tight control during its activation to achieve proper termination. (b) Gain of PHF20 recognizes p65 methylated at Lys221, and associates with p65. Such association may block a docking site for recruitment of PP2A into p65 that leads to persistent NF-κB response. Figure 7: Model for persistent activation of NF-κB by PHF20. It is known from the literature that NSD1 targets p65 for methylation on Lys218 and Lys221 residue functions to stabilize the formation of p65–DNA complex. p65 is also phosphorylated on Ser536 by various kinases, including IKKα, IKKβ or RSK1, which enhances its transactivation potential through recruiting histone acetyltransferase such as CBP and p300. ( a ) The recruitment of PP2A into phosphorylated p65 ensures that the NF-κB response maintains tight control during its activation to achieve proper termination. ( b ) Gain of PHF20 recognizes p65 methylated at Lys221, and associates with p65. Such association may block a docking site for recruitment of PP2A into p65 that leads to persistent NF-κB response. Full size image Previous studies have shown that the nuclear function of NF-κB is regulated through reversible methylation of its p65 subunit [32] , [39] . The methylation of p65 at Lys residues by methyltransferase Set9 or NSD1 was restricted to the nucleus, and is required for the expression of a subset of NF-κB target genes. Nevertheless, how this methylation, especially this that affects nuclear NF-κB proteins such as p65, is controlled and regulated is a question that remains yet largely unresolved. Given several protein domains, such as Tudor, Chromo, MBT and PHD domain, that have been identified as methylated lysine binding domains [40] , [41] , it has been hypothesized that these proteins may contribute to p65 methylation-dependent NF-κB activation. In this study, we showed that overexpression of a Tudor domain-containing protein, PHF20, results in a persistent p65 phosphorylation in the nucleus as well as in NF-κB-DNA binding. Such findings thus indicate that PHF20 functions as a transcriptional activator of NF-κB in the nucleus. This interpretation was further supported by the observations that (i) PHF20 expression was exclusively localized within the nucleus in cells and glioma tissues, and (ii) PHF20 induces persistent p65 phosphorylation only in nuclear fractions of TNF-treated cells. Most importantly, we found that PHF20 specifically interacts with p65 in a methylation (at the site of K221)-dependent manner via the Tudor2 domain, and such interaction is clearly required for persistent p65 phosphorylation induced by PHF20. Such observations indicate that PHF20 functions through the recognition of K221 dimethylation of p65, thus revealing a previously unknown mechanism for p65 methylation-mediated NF-κB hyperactivation in the nucleus. In regard to the functional consequence of p65 methylation, it has been reported that demethylation of p65 by knocking down methyltransferase Set9 did not affect TNF-induced IκBα expression, while the expression of other TNF-induced NF-κB target genes (IP-10 and TNF) were almost completely impaired [39] . Similarly, TNF-induced transcription of MnSOD, TNF and CCL-20 was markedly reduced in cells pretreated with MTA, while induction of IκBα was not affected (data not shown). These discrepancies of transcriptional regulation between IκBα and other NF-κB target genes may have resulted from the recruitment of different co-activators that depends on the status of p65 methylation. Further experiments will be needed to fully understand the regulatory mechanism of PHF20 on the transcription of NF-κB target genes. On the other hand, PHF20 was found to be an immunogenic antigen in the serum of patients with some malignancies including glioblastoma [17] , [18] , [19] , [20] . In this sense, how PHF20 translocates from the nucleus to extracellular matrix is also a question that remains to be further studied. Given that PHF20 was overexpressed in gliomas, it is possible that PHF20-mediated constitutive NF-κB activation caused by proinflammatory cytokines in tumour microenvironment may result in tissue injury and/or cell death [42] , leading to the release of PHF20 from the nucleus to serum in these patients. Therefore, further in vivo experiments will be needed to elucidate the dynamic cellular distribution of PHF20. In addition, future prospective clinical studies with a large scale of patients is required to establish the association between the NF-κB activation status and the serum levels of PHF20, providing evidence for developing PHF20 as a biomarker for NF-κB activation in certain types of malignancies. A critical finding from this study demonstrates that PHF20 induces persistent p65 phosphorylation by interacting with Lys-methylated p65. An earlier study reported that purified recombinant PP2A dephosphorylate p65 through physical interaction with p65 in in vitro [36] . In this study, we established that interactions between p65 and PP2A occur in response to TNF treatment. As the kinetics of such interaction correlated well with that of p65 phosphorylation, it is highly likely that PP2A, when recruited to p65, is responsible for the termination of p65 phosphorylation. More importantly, we show that dimethylation of p65 at Lys221 is required for interaction with PHF20, which in turn prevents the recruitment of PP2A into p65 and the subsequent dephosphorylation. Such observations thus reveal a novel mechanism through which PHF20 promotes NF-κB activation. The implications of this study raise multiple queries that remain yet to be explored. It is currently unclear how this methylation-dependent interaction of PHF20 and p65 functions to block the recruitment of PP2A. One of the possibilities is that interaction of PHF20 with methylated Lys221 within the loop structure of p65 may change the conformation of the loop and in turn block PP2A from accessing p65, as illustrated in Fig. 7 . Therefore, it is an open issue to clarify the structural basis for the dynamic interactions between PHF20 and methylated p65, and to fully understand the precise mechanisms through which PHF20 controls p65 phosphorylation. Antibodies and reagents All commercial antibodies and reagents were purchased from the following resources: anti-phospho-Ser/Thr PKB substrate (#9611, 1:1,000 dilution), anti-PKB (#9272, 1:1,000 dilution), anti-PHF20 (#39340, 1:1,000 dilution), anti-phospho-IκBα (#9246, 1:1,000 dilution), anti-IκBα (#9242, 1:1,000 dilution), anti-phospho-p65 (#3033, 1:1,000 dilution), anti-phospho-ERK1/2 Thr202/Tyr204 (#9101, 1:1,000 dilution), anti-phospho-JNK (#9251, 1:1,000 dilution), anti-myc (#2272, 1:2,000 dilution) and anti-acetyl-p65-Lys310 (#3045, 1:500 dilution) antibodies were from Cell Signaling Technology; anti-RIP1 (sc-7881, 1:1,000 dilution), anti-IKK-β (sc-7330, 1:1,000 dilution), anti-IKKγ (sc-8330, 1:1,000 dilution), anti-ERK (sc-94, 1:1,000 dilution), anti-JNK (sc-7345, 1:1,000 dilution), anti-p65 (sc-8008, 1:1,000 dilution), anti-p50 (sc-114, 1:1,000 dilution), anti-Xpress (sc-499, 1:2,000 dilution), anti-HA (sc-805, 1:2,000 dilution) and anti-SP1 (sc-59, 1:1,000 dilution) were from Santa Cruz Biotechnology Inc.; anti-actin (A2066, 1:2,000 dilution) and anti-flag (F3165, 1:1,000 dilution) antibodies, bacterial LPS, teb , etoposide, 5′-deoxy-5′-methylthioadenosine (MTA) were from Sigma-Aldrich; anti-p84N5 was from GeneTex; anti-PP2A catalytic subunit was from BD Biosciences; recombinant TNF and IL-1β were purchased from R&D Systems. Protein A and G-sepharose were purchased from Amersham Pharmacia Biotech; GST-IκBα (residues 1–54) were expressed and purified from Escherichia coli as described previously [43] . teb -inducible expression plasmid construction An ecdysone agonist, teb -dependent gene induction system, has become widely used in generating transgenic animals [44] . To develop easier and more versatile usage of the system in the mammalian cell, we combined the discrete driver and effector vectors into a single plasmid with several modifications, and designated the modified vector, termed as pEUI. After pEUI was digested with Eco RI, PCR product of PHF20 (WT or S291A) was introduced by EZ cloning core kit (Enzynomics, Korea). The detailed manuscript about the pEUI vector is under preparation. Immnunoblot analysis and immunoprecipitation After treatment as described in the figure legends, cells were collected and lysed in M2 buffer (20 mM Tris, pH 7.6, 0.5% NP-40, 250 mM NaCl, 3 mM EDTA, 3 mM EGTA, 2 mM dithiothreitol (DTT), 0.5 mM phenylmethyl sulphonyl fluoride, 20 mM β-glycerol phosphate, 1 mM sodium vanadate and 1 μg ml −1 leupeptin). Cell lysates were fractionated by SDS–polyacrylamide gel electrophoresis (SDS–PAGE) and visualized by enhanced chemiluminescence, according to the manufacturer’s instruction (Amersham). For immunopreciptation assays, the lysates were mixed and precipitated with the relevant antibody and protein G-A agarose beads by overnight incubation at 4 °C. The beads were washed three times with M2 buffer, and the bound proteins were resolved in 10% SDS–PAGE for immunoblot analysis. IKK kinase assay After treatments as described in the figure legends, cells were collected and lysed in M2 buffer. Whole-cell extracts were immunoprecipitated with an anti-IKKγ antibody, and protein A agarose beads for overnight. The beads were washed with lysis buffer, and kinase assay was then performed in complete kinase assay buffer (20 mM HEPES at pH 7.5, 20 mM β-glycerol phosphate, 10 mM MgCl 2 , 1 mM DTT, 10 mM PNPP, 50 μM sodium vanadate and 20 μM ATP) with the addition of [γ- 32 P]-ATP and 1 μg of GST–IκBα (1–54), as a substrate. After 20 min at 30 °C, sample buffer was added and proteins were resolved in 12% SDS–PAGE, and phosphorylated substrates were visualized by autoradiography. Quantitative real-time PCR analysis After the total RNA was extracted from cells using a TRIZOL reagent (Life Technologies Inc.), the oligo(dT)-primed complementary DNA was used for the reverse transcription of the purified RNA. The amount of transcript of the genes of interest was measured by real-time quantitative RT–PCR assay using the SYBR Green detection (Applied Biosystems, Carlsbad, CA). All reactions were independently repeated at least three times to ensure the reproducibility of the results. Primer sequences are listed in Supplementary Table S1 ). Luciferase reporter assays 293/IL-1R/TLR4, HEK293 and HeLa cells were co-transfected with p2xNF-κB-Luc, pRSV-β galactosidase, with or without various amounts of flag–PHF20, Xp-PHF20 expression vector or Ad–flag–PHF20 as indicated in the figure legends. For GAL4 one-hybrid system, HEK293 cells were co-transfected with GAL4–p65, GAL4-driven reporter (GAL4-tk-Luc), and with or without various amounts of flag–PHF20 expression vector. Twenty-four hours after transfection, cells were treated with TNF (15 ng ml −1 ) for additional 6 h, and luciferase activities in these cells were measured using a luciferase assay kit (Promega; Madison, WI, USA). Luciferase activity was normalized relative to β-galactosidase activity of each sample. Electrophoretic mobility shift assay Nuclear extracts for Electrophoretic mobility shift assay were prepared from HeLa cells as described previously [45] with minor modification. For binding reaction, 5 μg of nuclear extract was incubated at room temperature for 20 min with reaction buffer containing 20 mM HEPES at pH 7.9, 50 mM KCl, 0.1 mM EDTA, 1 mM DTT, 5% glycerol, 200 μg ml −1 BSA and 2 μg of poly(dI-dC)·poly(dI-dC). Then the 32 P-labelled double-stranded oligonucleotide containing the binding consensus sequence of NF-κB (5′-GGCAACCTGGGGACTCTCCCTTT-3′) or AP-1 (5′-CGCTTGATGACTCAGCCGGAA-3′) was added to the reaction mixture for an additional 10 min. The reaction products were fractionated on a non-denaturating 6% polyacrylamide gel, which was then dried and subjected to autoradiography. Confocal imaging analysis HeLa cells were grown on glass coverslips and then infected with rAd–PHF20 or rAd–Lac. After 24 h, the cells were treated as indicated in figure legend and fixed in 4% paraformaldehyde at room temperature for 10 min. Cells were washed in cold PBS and permeablized with 0.2% Triton X-100, and incubated with rabbit anti-p65 antibody (1:400 dilution; Santa Cruz Biothenology). The PE-conjugated secondary antibody (1:400 dilution; BD Pharmingen) was used and mounted with Fluromount-G (Vector Laboratories), and visualized using a fluorescence microscopy (Olympus, FV1200). Tissue specimens and histological grading A total of 36 paraffin-embedded archived clinical glioma specimens, including WHO I–IV grade tumours, were histopathologically diagnosed at the Chungnam National University Hospital, Daejeon, Korea from 2007–2011. The study was approved by the Hospital Institutional Review Board (approval number 07–21) according to the Declaration of Helsinki, and written informed consent was obtained from each patient by research team before surgery. According to the WHO classification, gliomas were classified into four grades, including grade I (2/36), grade II (4/36), grade III (8/36) and grade IV (22/36), respectively. No patients had received preoperative radiation therapy. Immunohistochemcal staining Immunohistochemical staining was performed using rabbit polyclonal anti-PHF20 (Santa Cruz Biotechnology Inc.) and anti-p-p65 (Abcam, UK) antibodies and EnVision-HRP detection system (DakoCytomation, Carpinteria, CA, USA) according to the manufacturer’s instruction. Paraffin sections (3 μm) were cut from gliomas, and deparaffinized in xylen and rehydrated in graded alcohol. After antigen retrieval by heating in a pressure cooker in target retrieval solution for 4 min, tissue sections were treated with 3% hydrogen peroxide for 10 min to block endogenous peroxidases. The sections were then incubated overnight at 4 °C with anti-PHF20 (1:80) and anti-p-p65 (1:50) antibodies diluted with background reducing diluents (S0809; Dako Cytomation). Slides were then incubated with EnVision reagent for 30 min, followed by 3,3′-diaminobenzidine chromogen for 5 min, counterstained with Meyer’s hematoxylin and mounted. Exclusion of the primary antibody during immunostaining was used as a negative control. Evaluation of immunohistochemical staining The immunohistochemical staining results were evaluated by two independent pathologist (J.M.K. and S.-M.H. ), who were blinded to patient’s clinocopathological details. Nuclear expression for the PHF20, and nuclear or cytoplasmic expression for the p-p65 were considered as positive cells. The immunohistochemical staining was categorized according to a scoring method based on the staining intensity (score 0, no staining intensity; score 1, weak staining intensity; score 2, intermediate staining intensity; and score 3, strong staining intensity). In the case of heterogenous staining within the samples, the respective higher score was chosen if >50% of the cells showed higher staining intensity. Immunofluorescent staining After having deparaffinized and hydrated with the same protocol used in immunohistochemistry, tissue specimens were incubated with the primary rabbit polyclonal anti-PHF20 (1:80) and mouse monoclonal anti-p-p65 (1:50) antibodies overnight at 4 °C. The sections were further incubated in a mixture of FITC- and Cys3-conjugated secondary antibodies, donkey anti-rabbit and goat anti-mouse IgG, for 1 h at room temperature, respectively. Each incubation step was followed by four 5 min rinses in PBS, and final tissue sections were mounted in PBS and analysed by fluorescence microscopy (Olympus, FV1200). Quantification of immunoreactive cells were performed by counting the number of positive cells at least 15 fields from each sample using Image J Colocalization Plugin software (version 1.43). Statistical analysis Data are expressed as the mean±s.e. from at least three separate experiments performed in triplicate. The differences between groups were analysed using Student’s t -test, and a P- value <0.05 was considered statistically significant. Statistical analyses were carried out using SPSS software ver. 13.0 (SPSS Inc., Chicago, IL). For statistical analysis of immunohistochemical staining intensity, group comparisons of categorical variables were evaluated using the χ 2 test or linear-by-linear association. Additional methods Information on the construction of plasmid and adenovirus, cell culture, adenovirus infection and transfection is available in the Supplementary Methods . How to cite this article: Zhang, T. et al. PHF20 regulates NF-κB signalling by disrupting recruitment of PP2A to p65. Nat. Commun. 4:2062 doi: 10.1038/ncomms3062 (2013).